Gold peroxide complexes and the conversion of hydroperoxides into gold hydrides by successive oxygen-transfer reactions Gold catalysts are widely studied in chemical and electrochemical oxidation processes. Computational modelling has suggested the participation of Au–OO–Au, Au–OOH or Au–OH surface species, attached to gold in various oxidation states. However, no structural information was available as isolable gold peroxo and hydroperoxo compounds were unknown. Here we report the syntheses, structures and reactions of a series of gold(III) peroxides, hydroperoxides and alkylperoxides. The Au–O bond energy in peroxides is weaker than in oxides and hydroxides; however, the Au–OH bond is also weaker than Au–H. Consequently Au–OH compounds are capable of oxygen-transfer generating gold hydrides, a key reaction in a water splitting cycle and an example that gold can react in a way that other metals cannot. For the first time it has become possible to establish a direct connection from peroxides to hydrides: Au–OO–Au→Au–OOH→Au–OH→Au–H, via successive oxygen-transfer events. Gold-based oxidation catalysts have been the subject of detailed investigations for over 20 years, ever since the first report of CO oxidation by supported gold nanoparticles [1] , [2] , [3] , [4] . The mode of oxygen activation remains unclear, not least as Au–O bonds are thought to be intrinsically weak and in general thermally unstable [5] , and the surfaces of gold catalysts adsorb O 2 only to a very limited extent [6] . It has been proposed that negatively charged gold nanoclusters facilitate O 2 adsorption by electron transfer to give surface superoxo-like species [4] , [5] , [6] , [7] , [8] , [9] , [10] , [11] , [12] , whereas Gates and co-workers [13] , and Hutchings et al . [14] , showed that high-activity gold catalysts for CO oxidation contain species in higher oxidation states (Au + , Au 3+ ). A very recent study postulated that Au 3+ peroxides and oxides are key intermediates in the electrochemical water splitting on gold electrodes [15] . A number of computational studies modelling oxidation reactions envisage the formation and interconversion of species with Au–O–O–Au, Au–OOH and Au–O–Au linkages [16] , [17] , [18] . To-date, there is, however, very little precise information available on the structures and bonding of such species; and although a number of gold oxo and hydroxo complexes have been reported [5] , such as the well-known cations [(LAu) 3 (μ-O)] + and [(LAu) 2 (μ-OH)] + (L=phosphine or carbene) [19] , [20] , [21] , [22] or the gold(III) oxo compounds [{(C^N^N)Au} 2 (μ-O)] 2+ and [(bipy) 2 Au 2 (μ-O) 2 ] 2+ (where C^N^N represents a tridentate cyclometallated 6-benzyl-2,2′-bipyridyl and bipy a substituted 2,2′-bipyridyl [23] , [24] , [25] , [26] , [27] , [28] , [29] , [30] , [31] ), to the best of our knowledge isolable peroxo, hydroperoxo and alkylperoxo complexes of gold (in any oxidation state) were unknown. We found recently that C^N^C pincer ligands based on the dianionic 2,6-diphenylpyridine framework are capable of stabilizing a number of novel gold(III) compound types [32] , [33] , including the first examples of gold(III) hydrides and olefin complexes [34] , [35] . Given the importance of oxygen ligands in oxidations as well as water cleavage reactions, we decided to explore the reactivity of such gold(III) pincer complexes towards oxygen ligands, including possible Au–O↔Au–H interconversions. We report here the formation and structures of a series of gold(III) compounds with O 2− , O 2 2− , HOO − and ROO − ligands, the nature of the Au–O bond in these compounds and their reactivity as oxidants, and we show that, unlike other metal hydroxides, a gold(III) hydroxide is readily converted into the corresponding gold hydride by oxygen-transfer, a step relevant to the water splitting cycle. Synthesis and characterization The reaction of the pincer complex (C^N^C)AuOH ( 1 ) [31] {(C^N^C)=[2,6-(C 6 H 3 t Bu-4) 2 pyridine] 2− } with t -butyl hydroperoxide in toluene at room temperature results in water elimination and formation of (C^N^C)AuOO t Bu ( 2 ), which was isolated as yellow crystals. An analogous reaction of 1 with an excess of 30% aqueous hydrogen peroxide in toluene rapidly leads to the precipitation of the hydroperoxide 3 , which was isolated as a yellow powder ( Fig. 1 ). Unlike 1 , compound 3 is only sparingly soluble in toluene. Although the 1 H NMR spectra of 1 and 3 are very similar, freshly prepared samples of 3 show an OH resonance at δ 8.26 (CD 2 Cl 2 ), which is not detectable for the hydroxide 1 . Over longer periods of time in CD 2 Cl 2 or THF solutions, the 1 H NMR pattern transforms into that of a new compound, identified as the bridging peroxide (C^N^C)AuOOAu(C^N^C) ( 4 ), which can be isolated as yellow crystalline blocks. The condensation is quite facile and recrystallization attempts of 3 repeatedly gave 4 instead. The condensation reaction is, however, reversible, and keeping 4 in water-saturated CD 2 Cl 2 solutions regenerated 1 and 3 . Treatment with dry solvents (acetone or THF) also induces the dehydration of the hydroxide 1 to give the bridging oxide complex 5 . The process is reversible, and exposure of 5 to moisture regenerates 1 . 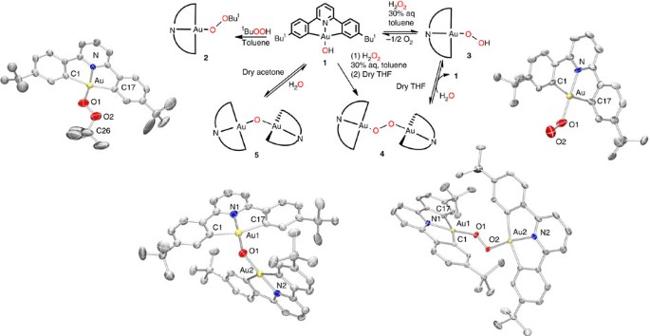Figure 1: Syntheses pathways of gold(III) peroxide and oxide complexes. Synthesis pathways showing the molecular structures of (C^N^C)AuOOtBu (2), (C^N^C)AuOOH (3), (C^N^C)AuOOAu(C^N^C) (4) and (C^N^C)AuOAu(C^N^C) (5) determined by X-ray diffraction. Ellipsoids are set at 50% probability. Hydrogen atoms are omitted for clarity. Figure 1: Syntheses pathways of gold(III) peroxide and oxide complexes. Synthesis pathways showing the molecular structures of (C^N^C)AuOO t Bu ( 2 ), (C^N^C)AuOOH ( 3 ), (C^N^C)AuOOAu(C^N^C) ( 4 ) and (C^N^C)AuOAu(C^N^C) ( 5 ) determined by X-ray diffraction. Ellipsoids are set at 50% probability. Hydrogen atoms are omitted for clarity. Full size image Unlike the hydroperoxide 3 , the tert -butylperoxide 2 and bridging peroxide 4 were found to be remarkably temperature stable. Heating THF solutions of 2 and 4 for 16 h at 60 °C leaves the compounds unchanged. Complexes 2 and 4 are also stable to ambient laboratory light giving no obvious signs of decomposition. Alternative synthesis protocols have been described for late transition metal peroxides involving direct O 2 insertions into metal-hydrogen [36] , [37] , [38] , metal-carbon [39] , [40] or metal-metal [41] bonds. However, these insertion routes proved to be unsuitable for the synthesis of the gold peroxides, and the reaction of the gold(III) hydride (C^N^C)AuH or the gold(II) dimer (C^N^C)Au–Au(C^N^C) [34] with 1 atmosphere of dioxygen under either thermal or photolytic conditions failed to give 3 or 4 , respectively. The O–O stretching vibration of peroxides 2 – 4 was examined by infrared (IR) spectroscopy. The IR spectrum of the hydroperoxide 3 is very similar to the hydroxide 1 but shows an additional band at 825 cm −1 (ref. 42 ), while the tert -butylperoxide 2 and the (μ-κ 1 :κ 1 -peroxo)digold complex 4 show three vibrational modes in the O–O stretching region, at 831, 844, 878 and 823, 828 and 844 cm −1 , respectively. For comparison, the O–O stretching frequency in H 2 O 2 is observed at 866 cm −1 (ref. 43 ), while a study on gold nanocluster catalysts by Yeo et al . [44] assigned a Raman band at 820 cm −1 to a surface-bound OOH species. The solid-state structures of 2 – 5 were determined by X-ray diffraction ( Fig. 1 ). Pertinent geometric parameters are collected in Table 1 . All complexes have Au–O distances of 1.971(4)–2.092(8) Å. The O–O bond distances in 2 and 4 (1.416(6)–1.448(4) Å) are within the typical range of distances recorded for coordinated peroxo moieties [36] , [37] , [38] , [39] , [40] , [41] and are closely comparable to that in H 2 O 2 . The oxide 5 has a bent structure, with an Au–O–Au angle of 113.5(2)°, as expected for an sp 3 -hybridized O atom. The results indicate negligible Au–O π-interactions; this aspect was subsequently confirmed by density functional theory (DFT) calculations ( vide infra ). Table 1 Comparison of geometric parameters of gold(III) peroxide and oxide complexes. Full size table The peroxide complexes readily react with electrophiles. For example, 2 oxidized acetaldehyde to acetic acid, which then forms (C^N^C)AuOAc ( 9 ), as confirmed by its independent synthesis, whereas 4 reacts with Me 3 SiBr to give (C^N^C)AuBr and a 2:1 mixture of Me 3 Si–OO–SiMe 3 and (Me 3 Si) 2 O. The attempted formation of a superoxo complex by reacting (C^N^C)Au(O 2 CCF 3 ) with KO 2 in a toluene/THF mixture (1:1) under an atmosphere of dioxygen led to the isolation of the crystallographically characterized furanolato complex (C^N^C)AuO(C 4 H 7 O) 10 as a product of THF oxidation ( Supplementary Fig. S1 ); this product was not formed in the absence of O 2 (see Supplementary Methods ). Oxygen-transfer reactions The ability of compounds 2 – 5 to act as oxidizing agents was tested using P( p -tolyl) 3 as reductant. Treating the hydroperoxide 3 with the phosphine in CD 2 Cl 2 solutions instantly led to the disappearance of the peroxo OOH resonance ( δ 8.26) and formation of O=P( p -tolyl) 3 and 1 , as observed by 1 H and 31 P{ 1 H} NMR spectroscopy. Similarly, treatment of the tert -butylperoxide 2 with one equivalent of phosphine leads to the formation of the phosphine oxide together with (C^N^C)AuO t Bu ( 6 ) ( Fig. 2 ). The reaction was found to be much slower than in the case of 3 and full conversion was only reached after 16 h. The identity of 6 was confirmed by its independent synthesis. 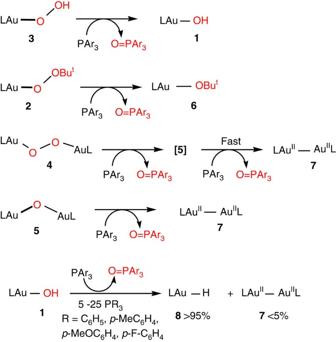Figure 2: Oxygen-transfer reactions of gold complexes. L represents the dianionic C^N^C ligand shown inFig. 1. Ar=p-tolyl. Figure 2: Oxygen-transfer reactions of gold complexes. L represents the dianionic C^N^C ligand shown in Fig. 1 . Ar= p -tolyl. Full size image The binuclear peroxide complex 4 in CD 2 Cl 2 oxidizes P( p -tolyl) 3 more slowly, with quantitative formation of O=P ( p -tolyl) 3 after 36 h. After 16 h, the reaction mixture showed a number of gold products, including 4 (21%), (C^N^C)AuCl (17%) and the gold(II) dimer (C^N^C)AuAu(C^N^C) ( 7 ) (25%), as well as other unidentified products. Interestingly, the peroxide 4 and the gold(II) complex 7 co-exist in solution, that is, the peroxide is unable to oxidize Au(II) to the Au(III) oxide 5 . We assume the reaction of 4 with phosphines proceeds by stepwise O-abstraction, to give first the oxide 5 . However, monitoring the reaction by 1 H NMR spectroscopy failed to show traces of 5 , which suggests that the second reduction step to gold(II) is fast. The formation of Au(II) from the Au(III) oxide was confirmed independently by treating 5 with P( p -tolyl) 3 which cleanly gives 7 . The oxygen-transfer reactions of 1 – 5 are summarized in Fig. 2 . Hydroxide to hydride conversion Carrying out the reduction of the hydroperoxide 3 with an excess of phosphine suggested the formation of an unexpected product, the hydride LAuH 8 , which was readily identified by its high-field 1 H NMR signal at δ −6.5 (in CD 2 Cl 2 ). The same was observed when (C^N^C)AuOH was reacted with an excess of phosphine. The formation of a gold hydride from a hydroxide was of interest as it represents a key step in a water splitting cycle. The cleavage of water into hydrogen and oxygen remains a highly desirable goal in the search for alternatives to fossil fuels but continues to pose significant challenges [45] . Efforts to construct catalytic cycles for water cleavage rely on a detailed understanding of each mechanistic step, and for catalysts based on well-defined coordination complexes a number of mechanisms are operative [46] , [47] , [48] . For metals that can readily alter their oxidation states and undergo oxidative additions, the formation of a metal hydrido-hydroxide M(H)(OH) is a key step, as realized recently by Milstein et al . using ruthenium pincer complexes [M=2,6-C 5 H 3 N(CH 2 PBu t 2 )(CH 2 NEt 2 )Ru] [49] . On the other hand, an alternative and potentially simpler pathway is available that does not require changes in oxidation states ( Fig. 3 ). This cycle involves the reaction of a metal cation with water to give a metal hydroxide. However, the key step in this scenario is the conversion of the metal hydroxide into a metal hydride. For most metals, the hydroxides are thermodynamically more stable than the hydrides, so that the M–OH→M–H transformation is not possible without an external hydride donor. The reaction of a metal hydroxide M–OH generating a metal hydride by O abstraction has to the best of our knowledge not previously been observed. 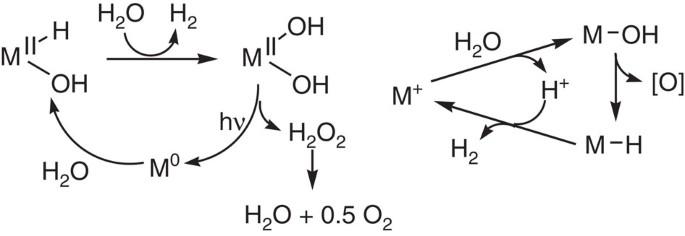Figure 3: Mechanisms of metal-mediated water cleavage. Although for ruthenium a redox mechanism involving M0and MII(OH)2intermediates has been demonstrated48, for other metals a non-oxidative pathway of water cleavage can be envisaged that involves a hydroxide-to-hydride transition. Figure 3: Mechanisms of metal-mediated water cleavage. Although for ruthenium a redox mechanism involving M 0 and M II (OH) 2 intermediates has been demonstrated [48] , for other metals a non-oxidative pathway of water cleavage can be envisaged that involves a hydroxide-to-hydride transition. Full size image A side reaction in the formation of (C^N^C)AuH from (C^N^C)AuOH is the Au(II) compound 7 ; this is, however, suppressed in a non-polar solvent such as toluene. The kinetics and mechanism of the oxygen-transfer from 1 was explored in the temperature interval from −10 to −55 °C. The reaction of 1 with an excess of P(C 6 H 4 X-4) 3 (X=H, Me, OMe, F) (5–25 molar equivalents) in toluene yields (C^N^C)AuH ( 8 ) with high selectivity (see box in Fig. 2 ). As gold complexes can be light sensitive, and in order to suppress possible radical side reactions, all reactions were conducted in the dark. To gain more insight into the reaction mechanism, the kinetics of the formation of 8 were followed by 1 H NMR spectroscopy (see Supplementary Figs S2–S6 , Supplementary Table S1 and Supplementary Methods ). The reaction is first-order in both gold and phosphine, −d[ 1 ]/d t = k [ 1 ][PR 3 ]. An Eyring plot over the temperature interval of −50 to −10 °C gave the activation parameters of the reaction as Δ H ‡ =−35.0(7) kJ mol −1 and Δ S ‡ =−105.7(2) J mol −1 K −1 (see Supplementary Figs S7–S9 ). The negative value of Δ S ‡ suggests that the reaction proceeds via an associative mechanism in the transition state. The origin of the oxygen in the phosphine oxide was established using (C^N^C)Au- 18 OH ( 1 - 18 O ). In the IR spectrum, the 18 OH vibration of 1 - 18 O is shifted to lower energy by 20 wavenumbers, to 3460, cm −1 . Mass spectrometric analysis showed the formation of 18 O=P( p -tol) 3 as the predominant product. The reaction of the deuterated complex (C^N^C)AuOD ( 1- d 1 ) with P( p -tol) 3 at 253 K resulted in a kinetic isotope effect k H / k D =1.45 ([(C^N^C)AuOH(D)] 0 :[P( p -tol) 3 ] 0 =1:10.8; k obs {(C^N^C)AuOH}=8.07(6) × 10 −4 s −1 , k obs {(C^N^C)AuOD}=5.49(3) × 10 −4 s −1 ) (see Supplementary Fig. S10 ). A KIE of this magnitude is consistent with the involvement of an O–H bending mode in the rate determining step [50] . The electronic effect of the rate of hydride formation was explored by a Hammett correlation using phosphines with electron withdrawing and donating p -substituents [51] . There is a strong influence ( ρ =−3.15, R 2 =0.94), with electron-donating groups such as Me or OMe substantially increasing the reaction rates (see Supplementary Figs S11, S12 and Supplementary Table 1 ). The negative ρ value (−1.05 per aryl ring) suggests that positive charge is built on the reaction centre and is in good agreement with a zwitterionic transition state. The reaction rates are insensitive to the presence of radical inhibitors. No significant effect on the rate constants was observed when the reaction of (C^N^C)AuOH with P( p -tol) 3 was carried in the presence or absence of TEMPO as radical scavenger (TEMPO=2,2,6,6-tetramethyl-1-piperidyl- N -oxide). Galvinoxyl was found to react with the hydride 8 quantitatively giving 7 . This implies that galvinoxyl is capable of H-abstraction from (C^N^C)Au–H while TEMPO is not. As the bond-dissociation energy (BDE) of TEMPOH is 291.34 kJ mol −1 , while the BDE of galvinoxyl-H is 328.7±2.1 kJ mol −1 , this provides an estimate of the Au–H bond energy between these two values, which was confirmed by DFT calculations. Quantum-chemical calculations The structures and bonding of these complexes was further investigated by computational modelling using DFT methods (see Supplementary Data 1 ). Optimization of the gas phase geometries of compounds 1 – 5 allowed calculation of Au–O and O–O bond energies ( Table 2 ). The Au–O bonds in the peroxides are significantly weaker than on the gold(III) oxide and hydroxide. Table 2 Calculated bond energies of gold(III) peroxide and oxide complexes. Full size table The O–O bonds weaken with increasing electron donation of the substituents. Similar effects were found for the O–O bond strengths in the series H 2 O 2 >MeOOH>MeOOMe (204, 186 and 158 kJ mol −1 , respectively) [52] , [53] . A consideration of the molecular orbitals shows that the HOMOs do not show a consistent Au–O bonding component, while the HOMO-1 orbitals show a variety of out-of-phase relationships between the oxygen lone pairs and the gold d -orbitals, that is, the interaction are anti-bonding ( Fig. 4 ). This confirms the weak π-interactions between the metal and the oxygen ligands that was already suggested by the acute Au–O–Au and Au–O–O angles in the solid-state structures. 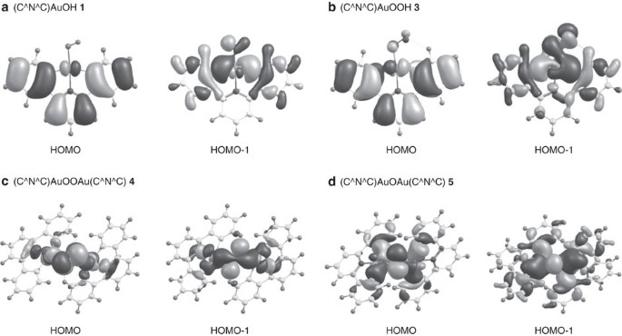Figure 4: HOMO and HOMO-1 orbitals. HOMO and HOMO-1 orbitals of complexes1(a),3(b),4(c) and5(d). The HOMO-1 diagrams show out-of-phase relationships between the gold-centred and the oxygen orbitals, most clearly seen in the case of1. Figure 4: HOMO and HOMO-1 orbitals. HOMO and HOMO-1 orbitals of complexes 1 ( a ), 3 ( b ), 4 ( c ) and 5 ( d ). The HOMO-1 diagrams show out-of-phase relationships between the gold-centred and the oxygen orbitals, most clearly seen in the case of 1 . Full size image The calculated trends in BDEs confirm the experimental findings: the Au–H bond is stronger than the Au–OH bond, whereas for isoelectronic Pt(II) complexes the opposite trend is observed ( Table 3 ). Table 3 Comparison of calculated and experimental bond-dissociation energies. Full size table Attempts to computationally identify an intermediate in the reaction of LAuOH with PR 3 , such as a 5-coordinate phosphine adduct of the gold complex or a zwitterionic intermediate [(C^N^C)Au ( δ −) (μ-OH)-PR 3 ( δ +) ] were unsuccessful. The results suggest a concerted mechanism for O-abstraction by PR 3 with simultaneous transfer of H from O to Au, as would be represented by a bending mode of the Au–O–H moiety as PR 3 approaches, in line with the observed modest kinetic deuterium isotope effect ( Fig. 5 ). 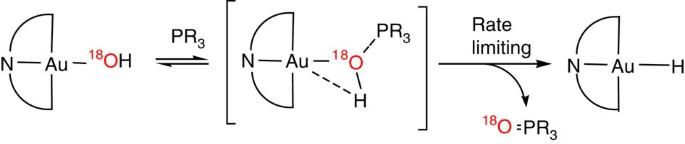Figure 5: Mechanistic pathway for the O-abstraction from gold(III) hydroxide by phosphines. The observed kinetic isotope effect and DFT calculations support a concerted oxygen-transfer mechanism. Figure 5: Mechanistic pathway for the O-abstraction from gold(III) hydroxide by phosphines. The observed kinetic isotope effect and DFT calculations support a concerted oxygen-transfer mechanism. Full size image The isolation, structural characterization and reactivity studies of this series of gold complexes highlights that in a suitable ligand environment gold peroxide complexes are readily accessible. However, it has also become evident that the Au–O bonds in peroxides are weaker than in oxides and hydroxides, that π-interactions in gold(III)–oxygen bonds are negligible, and that oxygen-transfer reactions are facile and well controlled. Surprisingly, even though the gold(II) complex supported by the pincer ligand used here possesses an unsupported Au–Au bond and its reaction with O 2 is calculated to be exothermic (−136 kJ mol −1 ), the complex fails to react with O 2 , and a route involving the hydroperoxide has to be used to access the anticipated binuclear gold peroxide. It remains to be established whether gold complexes can form side-on bonded O 2 compounds of the type familiar for Group 10 metals and postulated as surface species in gold nanocluster catalysts. Experimental observations, supported by bond energy calculations, demonstrate that only in the case of gold is the conversion of metal hydroxide M–OH into a hydride M–H thermodynamically favourable, enabling a key step of the water splitting cycle to proceed. The stability of the Au–H bond in (C^N^C)AuH is in part a consequence of the C^N^C pincer ligand framework and the weak trans influence exercised by the pyridine donor. Oxygen-transfer from the gold hydroxide to phosphines proceeds in a concerted fashion, with bending of the O–H bond toward the metal as the phosphine approaches. For the first time it could be shown that a succession of oxygen-transfer steps can provide a direct link between metal peroxides and metal hydride species, Au-OO-Au→Au-OOH→Au-OH→Au-H. General considerations Unless stated otherwise, manipulations were performed using standard Schlenk techniques under dry nitrogen or a Saffron Scientific glovebox. Anhydrous solvents were freshly distilled from appropriate drying agents. (C^N^C)AuOH {(C^N^C)=2,6-(C 6 H 3 Bu t -4) 2 -pyridine dianion} was prepared using literature methods. Additional experimental details can be found in the Supplementary Information . Synthesis of (C^N^C)AuOO t Bu (2) (C^N^C)AuOH ( 1 ) (200 mg, 0.36 mmol) and 4 Å molecular sieves were charged into a Schlenk flask and toluene (20 ml) was added. t BuOOH (5 M in dodecane, 100 μl, 0.5 mmol) was injected and the mixture was stirred at room temperature for 12 h. The mixture was filtered and the volatile components were removed in vacuo . The solid residue was washed with light petroleum (2 × 5 ml) and dried under vacuum to give 2 as a yellow powder (180 mg, 80%). Recrystallization from CH 2 Cl 2 : light petroleum (1:1) at−20 °C gave 2 as yellow blocks. 1 H NMR (300 MHz, CD 2 Cl 2 ) δ 7.91 (d, J =2 Hz, 2H, H 8 ), 7.79 (t, J =8.0 Hz, 1H, H 1 ), 7.49 (d, J =8 Hz, 2H, H 5 ), 7.38 (d, J =8 Hz, 1H, H 2 ), 7.28 (dd, J =8, 2 Hz, 2H, H 6 ), 1.40 (s, 9H, OOC Me 3 ), 1.36 (s, 18H, C 11 ) (see Supplementary Fig. S13 ). 13 C{ 1 H} NMR (75 MHz, CD 2 Cl 2 ) δ 170.80 (C 9 ), 164.41 (C 3 ), 154.96 (C 7 ), 145.45 (C 4 ), 142.42 (C 1 ), 130.65 (C 8 ), 124.82 (C 5 ), 124.36 (C 6 ), 116.30 (C 7 ), 79.68 (OO C Me 3 ), 35.75 (C 10 ), 31.33 (C 11 ), 26.49 (OOC Me 3 ). IR: 831, 844, 878 cm −1 . Anal. Calcd. (found) for C 29 H 36 AuNO 2 : C, 55.50 (55.59); H, 5.78 (5.80); N, 2.23 (2.34). Synthesis of (C^N^C)AuOOH (3) Under air, 1 (200 mg, 0.26 mmol) was dissolved in toluene (30 ml) and H 2 O 2 (30% aq, 82 μl, 0.52 mmol) was added. A yellow precipitate was immediately observed. The mixture was stirred for 30 min at room temperature, after which the supernatant was decanted and the yellow precipitate was washed with acetonitrile (5 ml) and light petroleum (5 ml) to afford 3 as a yellow powder (95.6 mg, 65%). Anal. Calcd. (found) for C 25 H 28 AuNO 2 : C, 53.54 (52.91); H, 4.94 (4.80); N 2.45 (2.35). The elemental analysis was carried out on as-precipiatetd material; recrystallization attempts lead to contamination with the peroxide 4 . 1 H NMR (300 MHz, CD 2 Cl 2 ) δ 8.26 (s, 1H, OO H ), 7.83 (t, J =8 Hz, 1H, H 1 ), 7.62 (d, J =2 Hz, 2H, H 8 ), 7.52 (d, J =8 Hz, 2H, H 5 ), 7.41 (d, J =8. Hz, 2H, H 2 ), 7.30 (dd, J =8, 2 Hz, 2H, H 6 ), 1.36 (s, 18H, H 11 ) (see Supplementary Fig. S14 ). 13 C data could not be obtained because of the degradation of (C^N^C)AuOOH in solution. IR: 825 cm −1 . Recrystallization from CH 2 Cl 2 : light petroleum (1:1) at +5 °C overnight gave 3 as yellow blocks, which were analysed by X-ray diffraction. Synthesis of (C^N^C)AuOOAu(C^N^C) (4) A solution of 3 (150 mg, 0.25 mmol) in dry THF (10 ml) was kept in the dark at room temperature. After 3 days, yellow crystalline blocks were observed. The supernatant was filtered off and the residue dried in vacuo , giving 4 as yellow crystals. An additional crop of crystals could be obtained by concentrating the mother liquor and leaving the solution to stand at room temperature. Total yield: 81 mg, 55%. The crystals obtained were suitable for X-ray diffraction. 1 H NMR (300 MHz, CD 2 Cl 2 ) δ 8.23 (d, J =2 Hz, 2H, H 8 ), 7.80 (t, J =8 Hz, 1H, H 1 ), 7.51 (d, J =8 Hz, 2H, H 5 ), 7.41 (d, J =8 Hz, 1H, H 2 ), 7.23 (dd, J =8, 2 Hz, 2H, H 6 ), 1.14 (s, 18H, H 11 ) (see Supplementary Fig. S15 ). 13 C{ 1 H} NMR (75 MHz, CD 2 Cl 2 ) δ 170.14 (C 9 ), 163.45 (C 3 ), 154.41 (C 7 ), 145.48 (C 4 ), 141.63 (C 1 ), 129.99 (C 8 ), 124.35 (C 5 ), 123.71 (C 6 ), 115.73 (C 7 ), 35.27 (C 10 ), 30.91 (C 11 ). IR: 823, 828, 844 cm −1 . Anal. Calcd. (found) for C 50 H 54 Au 2 N 2 O 2 : C 54.16 (54.00); H 4.91 (5.01); N, 2.53 (2.59). Synthesis of (C^N^C)AuOAu(C^N^C) (5) A solution of 1 (100 mg, 0.18 mmol) in dry acetone (20 ml) was stirred for 16 h at 60 °C. The resulting precipitate was collected and was washed with acetone (5 ml) and light petroleum (5 ml) to give 5 as a yellow powder (49 mg, 50%). Crystals suitable for X-ray diffraction were obtained by layering a dichloromethane solution of 5 with light petroleum at −25 °C. 1 H NMR (300 MHz, CD 2 Cl 2 ) δ 8.32 (d, 2.0 Hz, 2H, pyridyl), 7.77 (t, J =8.0 Hz, 1H, pyridyl), 7.50 (d, J =8 Hz, 2H, phenyl), 7.41 (d, 8.0 Hz, 2H, phenyl), 7.20 (dd, J =8, 2 Hz, 2H, phenyl), 1.08 (s, 18H, t Bu) (see Supplementary Fig. S16 ). 13 C{ 1 H} NMR (75 MHz, CD 2 Cl 2 ) δ 173.73 (C 9 ), 164.16 (C 3 ), 154.85 (C 7 ), 145.26 (C 4 ), 141.33 (C 1 ), 131.18 (C 8 ), 124.16 (C 5 ), 123.22 (C 6 ), 115.57 (C 7 ), 35.18 (C 10 ), 30.80 (C 11 ). Anal. calcd. for C 50 H 54 Au 2 N 2 O (found): C 54.95 (55.03); H 4.98 (5.09); N, 2.56 (2.66). Synthesis of (C^N^C)AuO t Bu (6) To (C^N^C)Au(O 2 CCF 3 ) (50 mg, 0.08 mmol) and 4 Å molecular sieves in a Schlenk tube was added a mixture of toluene and t BuOH (1:1, 10 ml). After stirring at room temperature for 12 h, the volatiles were removed in vacuo and the residue was extracted with dichloromethane (15 ml) and filtered. Removal of the solvent gave (C^N^C)AuO t Bu as a deep yellow powder (24 mg, 50%). 1 H NMR (300 MHz, CD 2 Cl 2 ) δ 7.99 (d, J =2 Hz, 2H, H 8 ), 7.78 (t, J =8 Hz, 1H, H 1 ), 7.49 (d, J =8 Hz, 2H, H 5 ), 7.39 (d, J =8 Hz, 2H, H 2 ), 7.27 (dd, J =8, 2 Hz, 2H, H 6 ), 1.49 (s, 9H, OC(C H 3 ) 3 ), 1.38 (s, 18H, H 11 ) (see Supplementary Fig. S17 ). 13 C{ 1 H} NMR (75 MHz, CD 2 Cl 2 ) δ 171.79 (C 9 ), 164.67 (C 3 ), 154.43 (C 7 ), 145.21 (C 4 ), 142.20 (C 1 ), 131.92 (C 8 ), 124.24 (C 5 ), 123.63 (C 6 ), 115.87 (C 2 ), 74.24 (O C Me 3 ), 35.41 (C 10 ), 34.84 (OC Me 3 ), 30.97 (C 11 ). Anal. calcd. (found) for C 29 H 36 AuNO: C 56.95 (56.90), H 5.93 (5.85), N, 2.29 (2.33). Synthesis of (C^N^C)AuOAc (9) A mixture of (C^N^C)AuCl (152 mg, 0.349 mmol) and AgOAc (45 mg, 0.384 mmol) in dichloromethane (100 ml) was stirred at room temperature for 36 h in the dark. The precipitate of AgCl was filtered off and volatiles were removed in vacuo to yield (C^N^C)AuOAc as a bright yellow powder (196 mg, 88%). 1 H NMR (300 MHz, CD 2 Cl 2 ) δ 7.85 (t, J =8 Hz, 1H, H 1 ), 7.54–7.45 (m, 4H, H 8 +H 5 ), 7.39 (d, J =8 Hz, 2H, H 2 ), 7.32 (dd, J =8.2, 2 Hz, 2H, H 6 ), 2.34 (s, 3H, OCOC H 3 ), 1.38 (s, 18H, H 11 ) (see Supplementary Fig. S18 ). 13 C{ 1 H} NMR (75 MHz, CD 2 Cl 2 ) δ 174.25 (O= C ), 169.50 (C 9 ), 165.21 (C 3 ), 155.22 (C 7 ), 144.56 (C 4 ), 143.15 (C 1 ), 129.80 (C 8 ), 124.82 (C 5 ), 124.37 (C 6 ), 116.24 (C 2 ), 35.23 (C 10 ), 30.86 (C 11 ), 22.36 (OCO C H 3 ). Anal. calcd. (found) for C 27 H 30 AuNO 2 : C 56.34 (56.45), H 5.67 (5.50), N 2.19 (2.31). Kinetics of O-abstraction from 1 with phosphines Stock solutions of 1 (14.4 mM), PR 3 (151 mM) and 18-crown-6 (internal standard, 300 mM) in toluene- d 8 were prepared. To a solution of 1 (0.5 ml, 14.4 mM, 7.2 μmol) in toluene- d 8 was added a solution of 18-crown-6 (20 μl, 300 mM, 6 μmol). The mixture was cooled at −78 °C. Under light exclusion an appropriate amount of a pre-cooled solution of (p-tolyl) 3 P (151 mM) was added. The NMR tube was briefly shaken before being inserted into the NMR probe, which was pre-cooled to the appropriate temperature. The reaction was monitored by 1 H NMR spectroscopy. Data points were collected at regular intervals (typically 120 s, with D1=1 s, AQ=5.3 s and NS=16 scans). Observed rates were determined under pseudo-first order conditions by monitoring the disappearance of the resonance of H 8 for 1 , ( δ =8.13), the increase of the resonance of H 8 for (C^N^C)AuH 8 ( δ =8.40) and aromatic proton signals for O=P( o -tolyl) 3 ( δ =7.79) versus the resonance of the internal standard ( δ =3.51) (see Supplementary Figs S19,S20 ). Spectra were integrated automatically using the multi_integ3 command in TopSpin and the baseline correction was done manually. For details see Supplementary Methods . Accession codes : The X-ray crystallographic coordinates for structures reported in this Article (see Supplementary Table 2 ) have been deposited at the Cambridge Crystallographic Data Centre (CCDC), under deposition numbers CCDC 936989 ( 2 ), CCDC 936992 ( 3 ), CCDC 936990 ( 4 ), CCDC 936991 ( 5 ), CCDC 936993 ( 9 ) (ref. 54 ). These data can be obtained free of charge from the Cambridge Crystallographic Data Centre via www.ccdc.cam.ac.uk/data_request/cif . How to cite this article: Roşca, D.-A. et al . Gold peroxide complexes and the conversion of hydroperoxides into gold hydrides by successive oxygen-transfer reactions. Nat. Commun. 4:2167 doi: 10.1038/ncomms3167 (2013).